Mouldable all-carbon integrated circuits A variety of plastic products, ranging from those for daily necessities to electronics products and medical devices, are produced by moulding techniques. The incorporation of electronic circuits into various plastic products is limited by the brittle nature of silicon wafers. Here we report mouldable integrated circuits for the first time. The devices are composed entirely of carbon-based materials, that is, their active channels and passive elements are all fabricated from stretchable and thermostable assemblies of carbon nanotubes, with plastic polymer dielectric layers and substrates. The all-carbon thin-film transistors exhibit a mobility of 1,027 cm 2 V −1 s −1 and an ON/OFF ratio of 10 5 . The devices also exhibit extreme biaxial stretchability of up to 18% when subjected to thermopressure forming. We demonstrate functional integrated circuits that can be moulded into a three-dimensional dome. Such mouldable electronics open new possibilities by allowing for the addition of electronic/plastic-like functionalities to plastic/electronic products, improving their designability. Conventional integrated circuits (ICs) built on silicon wafers are rigid and fragile. However, recently, flexible devices have been fabricated on polymer films [1] , [2] . In addition to flexibility, polymer materials exhibit plasticity or mouldability and can be permanently deformed into arbitrary shapes by applying mechanical force and heat. A variety of plastic products, ranging from those for daily necessities to electronics products and medical devices, are produced by such moulding techniques. However, neither the conventional semiconductor materials nor the electrodes/interconnections that comprise ICs can be moulded, owing to their poor stretchability and heat tolerance. Carbon nanotube (CNT) assemblies have excellent mechanical flexibility and stretchability as well as electric conductivity and heat tolerance. They have been used in various electronic and electromechanical devices, including flexible transparent conductive films [3] , [4] , [5] , thin-film transistors (TFTs) [6] , [7] , [8] , [9] , [10] , functional ICs [8] , [9] , [11] and electromechanical sensors [12] . Currently available carbon-based devices such as TFTs [13] , [14] , [15] , [16] usually exhibit limited flexibility and stretchability owing to the use of rigid metal electrodes and oxide insulators (such as Al 2 O 3 and SiO 2 , to name a few). Gate dielectrics made of polymers [17] and ionic liquids [18] have been introduced as alternatives; however, these usually result in high operating voltages and low operating speeds, respectively. In this study, we demonstrate fully transparent and extremely stretchable TFTs and ICs that can operate at low voltages with a thick polymer gate insulator, utilizing the field focusing effect. We also show that these devices are mouldable via an air-assisted thermopressure-forming technique. All-carbon TFTs and ICs We fabricated top-gate-type TFTs and ICs on a polyethylene naphthalate (PEN) substrate with a thickness of 125 μm. The active layer comprised a sparse network-like CNT thin film and the passive elements a dense 80-nm thick CNT thin film, with the dielectric and intermediate layers consisting of a 660-nm thick polymethyl methacrylate (PMMA) layer. We grew the CNTs using a floating-catalyst (aerosol) chemical vapour deposition technique [19] ; collected them on a membrane filter, while controlling the CNT density to the appropriate level by adjusting the collection time; transferred the CNT film onto the substrate; and patterned it using standard photolithographic and oxygen plasma etching processes [9] . The average diameters of CNTs were evaluated from the optical absorption spectrum to be 1.1 nm for the channel [9] and 1.4 nm for the electrodes and interconnections [5] . The CNT electrodes and interconnections exhibit a sheet resistance of ∼ 230 Ω sq −1 and a transparency of 85% at a wavelength of 550 nm after being chemically doped with HNO 3 for 1 min. As can be seen from Fig. 1a , the fabricated devices are fully transparent and flexible, with their transmittance being ∼ 10% lower than that of the PEN substrate and reaching up to ∼ 80% when 48% of the substrate is covered with the thick CNT film that forms the electrodes and the interconnections as shown in Fig. 1b . The colour map in the inset shows that the all-carbon ICs have less colour as compared with previously reported transparent devices based on oxides such as ZnO and indium tin oxide [13] , [20] . 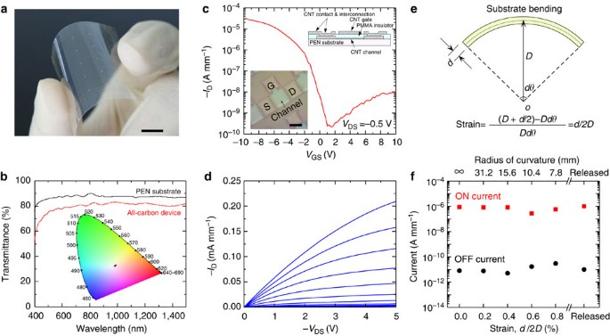Figure 1: Flexible and transparent all-carbon TFTs and ICs. (a) Photograph of an all-carbon device fabricated on a flexible PEN substrate (scale bar, 10 mm). (b) Optical transmittance of the PEN substrate (black line) and the device fabricated on the substrate (red line). Inset: plot showing the colour space (CIE 1931); the cross represents the colour white, and the black and red dots represent the colours of a bare PEN substrate and the all-carbon IC, respectively. (c) Transfer (ID−VGS) characteristics of an all-carbon top-gate TFT atVDS=−0.5 V.Lch=Wch=100 μm. Insets: optical micrograph of an all-carbon top-gate TFT array (bottom-left, scale bar, 100 μm) and a schematic showing the cross-section of the all-carbon device (top-right). (d) Output (ID−VDS) characteristics of all-carbon TFT.VGSwas varied from −10 to 0 V in 1-V steps. (e) Schematic showing a bent substrate. The radius of curvature,D,is measured from the point of origin,O, to the neutral axis of the substrate. The bending angle isdθ. The linear strain is given by the equation. (f) The ON and OFF currents of the all-carbon TFT for the different bending levels. Figure 1: Flexible and transparent all-carbon TFTs and ICs. ( a ) Photograph of an all-carbon device fabricated on a flexible PEN substrate (scale bar, 10 mm). ( b ) Optical transmittance of the PEN substrate (black line) and the device fabricated on the substrate (red line). Inset: plot showing the colour space (CIE 1931); the cross represents the colour white, and the black and red dots represent the colours of a bare PEN substrate and the all-carbon IC, respectively. ( c ) Transfer ( I D − V GS ) characteristics of an all-carbon top-gate TFT at V DS =−0.5 V. L ch = W ch =100 μm. Insets: optical micrograph of an all-carbon top-gate TFT array (bottom-left, scale bar, 100 μm) and a schematic showing the cross-section of the all-carbon device (top-right). ( d ) Output ( I D − V DS ) characteristics of all-carbon TFT. V GS was varied from −10 to 0 V in 1-V steps. ( e ) Schematic showing a bent substrate. The radius of curvature, D, is measured from the point of origin, O , to the neutral axis of the substrate. The bending angle is dθ . The linear strain is given by the equation. ( f ) The ON and OFF currents of the all-carbon TFT for the different bending levels. Full size image Figure 1c shows the transfer characteristics of an all-carbon top-gate TFT. The channel length ( L ch ) and channel width ( W ch ) are both 100 μm. The device exhibits p-type characteristics with a high ON/OFF ratio of >10 5 and the subthreshold voltage of 0.73 V dec −1 . The effective device mobility was 1,027 cm 2 V –1 s –1 , which was evaluated in the linear region at V DS =−0.5 V using the standard formula μ =( L ch / W ch )(1/ C )(1/ V DS )( dI D / dV GS ). Here, C was estimated using a rigorous model that takes into account the realistic electrostatic coupling between the sparse CNTs and the gate electrode [21] . The mobility of the fabricated all-carbon TFTs exceeds not only those previously reported for CNT TFTs [9] , [22] and low-temperature poly-Si TFTs [23] , [24] but also that reported for single-crystal Si metal–oxide–semiconductor field-effect transistors [25] . For C calculated using a parallel-plate model, that is, for C = ɛ / t ox , where ɛ is the dielectric constant of the gate insulator, the effective mobility is 321 cm 2 V –1 s –1 . Even for the high carrier mobility, the output saturation current density per unit device width (210 μA mm −1 at V DS =−5 V, Fig. 1d ) was still much smaller than conventional Si metal–oxide–semiconductor field-effect transistors. This is mainly due to the small gate capacitance composed by the thick PMMA gate insulator and low-density CNT channel. It is worth mentioning that the I D − V DS characteristics exhibit ohmic behaviour in the linear region as shown in Fig. 1d , suggesting a formation of good ohmic contacts between the CNT channel and CNT electrodes. As the all-carbon devices are made of CNTs and polymers, they exhibit better flexibility and stretchability compared with devices fabricated from rigid metals and oxide insulators. We performed the bending tests, in which the all-carbon devices were rolled, under various conditions, on cylinders having different diameters. When a substrate with a thickness ( d ) is bent with a radius of curvature ( D ) measured from the point of origin O to the natural axis of the substrate, the linear tensile strains of d /2 D is experienced by the outer surfaces of the devices as shown in Fig. 1e . The all-carbon TFTs exhibit only a small variation in the ON and OFF currents when subjected to bending strains of up to 0.8% as shown in Fig. 1f , thus demonstrating that the devices exhibited good flexibility. We fabricated all-carbon ICs, including inverters; 11- and 21-stage ring oscillators; NOR, NAND and XOR gates; and static random access memory (SRAM) cells. The CNT electrodes and PMMA insulators were similar to those of the all-carbon TFTs. The load for the logic gates is a gate-source-shorted all-carbon TFT. The channel width of the load TFTs is designed to be 50 μm, whereas that of the driver is 100 μm in order to adjust the thresholds of the logic gates. 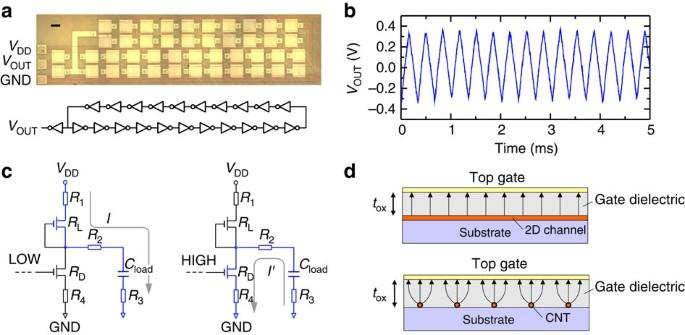Figure 2: 21-stage all-carbon ring oscillator. (a) Optical micrograph and circuit diagram (scale bar, 100 μm). (b) Oscillation waveform. (c) Schematic circuits showing charging (left) and discharging (right) processes in an inverter connected to the load capacitance. (d) Schematics showing the electric force lines in a 2D channel (top) and a sparse CNT channel (bottom). In the case of 2D channels found in conventional semiconductor TFTs, the electric force lines are uniformly distributed. On the other hand, in case of the sparse CNT thin film, in which the spacings between the CNTs are greater than the thickness of the gate insulator, the electric force lines are focused on the CNTs in the channel. Figure 2a,b , respectively, show the photograph and circuit diagram and the oscillation waveform for a 21-stage all-carbon ring oscillator, in which 21 inverters are connected in series and with which an additional output buffer is integrated, resulting in the device having 44 TFTs in total. The output voltage begins oscillating spontaneously at a V DD of −3 V. The oscillation frequency reaches a value of 3.0 kHz at a V DD of −5 V, and the delay time for each inverter is 7.9 μs per gate, which is shorter than that for the ring oscillators with Au interconnections that we had reported previously [9] . Although the parasitic resistances of the CNT electrodes and interconnections are higher than those of metals, they do not significantly influence the delay times because the RC delay in switching is primarily caused by the ON resistance of the TFTs. The oscillation frequency of the ring oscillator is determined by the total gate delay of the inverters in the circuit chain. The delay time ( τ ) of each inverter can be approximated by the product of the total series resistance and the load capacitance ( C load ) attributable to the gate of the inverter of the next stage. Thus, as shown in the simplified models in Fig. 2c . Here the resistance includes the resistances of the CNTs and the interconnections ( R 1 , R 2 , R 3 and R 4 ) and the ON resistances ( R L and R D ) of the TFTs. We estimated the resistances in the fabricated all-carbon devices to be R 1 ∼ 7 kΩ, R 2 ∼ 1.5 kΩ, R 3 ∼ R 4 ∼ 15 kΩ, R L ∼ 2 MΩ and R D ∼ 1 MΩ, respectively, showing that the delay time is mostly determined by the channel resistance. Figure 2: 21-stage all-carbon ring oscillator. ( a ) Optical micrograph and circuit diagram (scale bar, 100 μm). ( b ) Oscillation waveform. ( c ) Schematic circuits showing charging (left) and discharging (right) processes in an inverter connected to the load capacitance. ( d ) Schematics showing the electric force lines in a 2D channel (top) and a sparse CNT channel (bottom). In the case of 2D channels found in conventional semiconductor TFTs, the electric force lines are uniformly distributed. On the other hand, in case of the sparse CNT thin film, in which the spacings between the CNTs are greater than the thickness of the gate insulator, the electric force lines are focused on the CNTs in the channel. Full size image We also confirmed that the other functions of the ICs worked at V DD of −5 V ( Supplementary Fig. 1 ). It is worth mentioning that the various functions of the ICs could be tested at the fairly low voltage of −5 V even though a 660-nm thick polymer layer was used for the gate insulator in the TFTs. It is known that a thicker insulator usually leads to a higher operating voltage (tens of volts) in conventional Si-based TFTs and organic TFTs [26] , because the gate-to-channel capacitance necessary for charging the carriers in the channel decreases in inverse proportion to the thickness of the gate insulator for a conventional two-dimensional (2D) channel. However, for a sparse network-like CNT thin film in which the spacings between the CNTs are large compared with the thickness of the gate insulator, the electrostatic coupling between the nanotubes and the gate electrode is enhanced because the electric force lines are focused on the nanotubes, whose diameters are in the nanometre range, as shown in Fig. 2d . As a consequence, the gate-to-channel capacitance approximately becomes a function of log −1 ( t ), where t is the thickness of the gate insulator, leading to the gate-to-channel capacitance having a considerable value even for an increased gate insulator thickness, in contrast to what is noticed in 2D channels. On comparing the devices fabricated in this study with previously reported ones having inorganic gate insulators (Al 2 O 3 ; t ox : 40 nm; relative dielectric constant ( ɛ r ): 10) [9] , the equivalent oxide layer thickness ( t OX ε SiO 2 / ε r ) for the present devices, which use PMMA as the gate insulator ( t ox : 660 nm; ɛ r : 3.4), increases from 15.6 to 757 nm. Here, ɛ SiO2 is relative dielectric constant of SiO 2 . For this case, the gate capacitance of the parallel-plate capacitor decreases to be 2%, whereas the capacitance of the sparse CNT channel is 41.5% of the initial value, resulting in an increase in the gate effect by a factor of 20.8. The low-voltage operation of the fabricated ICs is attributable to the sparse network-like CNT film. The large gate-induced hysteresis typically observed in transfer characteristics of CNT transistors is one of the issues to be addressed. The present all-carbon TFTs exhibited relatively smaller hysteresis than previous CNT TFTs with a bottom gate structure [9] ( Supplementary Fig. S2 ). This is probably because the channel is covered with the PMMA gate insulator layer so as to decrease the amount of adsorbing ambient molecules such as water and oxygen causing hysteresis [27] , [28] , [29] . Although the width of hysteresis increased with sweep amplitude of V GS , in the range of an operation voltage of present ICs ( V DD =−5 V), the hysteresis is still small enough to secure the noise margin for the logic operation as will be shown later. Mouldability of all-carbon devices The unique compositions of the devices allows them to be deformed in a three-dimensional (3D) manner using extremely high strains, which are induced via moulding using an air-assisted thermopressure-forming technique. This technique is shown schematically in Fig. 3a . The planar substrate is heated and blown to form a dome-shaped structure ( Fig. 3b ). The all-carbon device, as well as the PEN substrate, is then stretched biaxially during the forming process as shown in Fig. 3c . The process does not cause the CNT films to crack or peel, and the channel width and length both increase from 100 to 112 μm, corresponding to biaxial tensile strains of 12% (25% increase in area). This is in sharp contrast to rigid materials such as metals, which generally break down for strains greater than 1% ( Supplementary Fig. S3 ). Moreover, the positions of upper layers such as the gate insulator and gate electrode did not shift relatively to the position of underlying drain/source and channel layers in the moulding process. The radii of curvature of the dome-shaped devices and the tensile strains induced in them can be controlled through the forming temperature as shown in Fig. 3d . 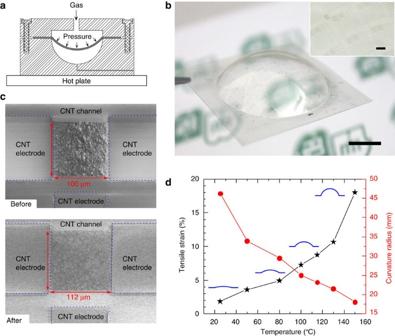Figure 3: Moulding of the all-carbon devices. (a) Schematic of the cross-section of the air-assisted thermopressure-forming apparatus. (b) Photograph of a dome-shaped all-carbon device (scale bar, 10 mm). Inset: magnified photograph (scale bar, 1 mm). (c) SEM images of the CNT channels and electrodes before and after the application of a biaxial tensile strain of 12% (scale bars, 100 μm). (d) Dependence on the forming temperature of the tensile strain and the corresponding radii of curvature. Figure 3: Moulding of the all-carbon devices. ( a ) Schematic of the cross-section of the air-assisted thermopressure-forming apparatus. ( b ) Photograph of a dome-shaped all-carbon device (scale bar, 10 mm). Inset: magnified photograph (scale bar, 1 mm). ( c ) SEM images of the CNT channels and electrodes before and after the application of a biaxial tensile strain of 12% (scale bars, 100 μm). ( d ) Dependence on the forming temperature of the tensile strain and the corresponding radii of curvature. 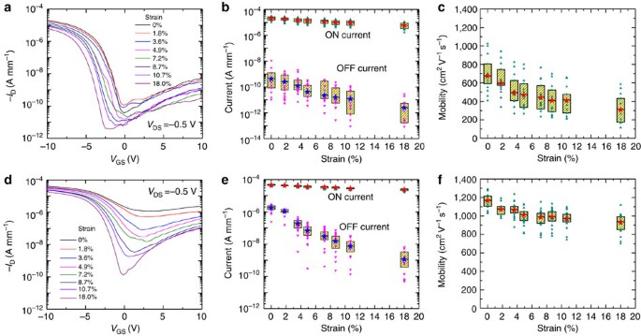Figure 4: Variation of property of all-carbon devices when subjected to moulding. (a–c) Transfer characteristics, ON and OFF currents, and mobilities of the all-carbon TFTs moulded under different conditions. The TFTs have a low-density channel, which leads to a high initial ON/OFF ratio.VDS=−0.5 V.Lch=Wch=100 μm. The currents are normalized to the same unit (A mm−1) because the channel dimensions increase after the moulding process. The ON and OFF currents and mobilities of 20 TFTs are plotted versus strain. The solid stars represent the median, and the upper and lower bands of the boxes correspond to the 75th and 25th percentiles, respectively, of the device population. (d–f) Transfer characteristics, currents and mobilities of the all-carbon TFTs moulded under different conditions. The TFTs have high-density channels, which lead to low initial ON/OFF ratios. Full size image Figure 4a–f show the variations in the static characteristics of the all-carbon TFTs for a series of biaxial tensile strains with values up to 18.0%. The detail of the uniformity in the device property is shown in Supplementary Fig. S4 . These TFTs were prepared using CNTs in two different densities; the lower density (0.67 CNTs μm −1 ) results in an initial ON/OFF ratio of ∼ 10 6 ( Fig. 4a ), whereas the higher one (1.34 CNTs μm −1 ) leads to an initial ON/OFF ratio of <10 2 ( Fig. 4d ). It is known that even if the metallic CNTs are incorporated in the channel in an amount of 30%, a high ON/OFF ratio can still be obtained by adjusting the density of the CNTs such that it is lower than the percolation threshold [30] . On increasing the strain, the ON currents decrease slightly in both devices as shown in Fig. 4b,e . Consequently, the median mobility decreases from 675 to 311 cm 2 V –1 s –1 for the lower CNT density ( Fig. 4c ) and from 1,168 to 935 cm 2 V –1 s –1 for the higher one ( Fig. 4f ). We could notice two distinct trends in the OFF currents of the two devices. The ON/OFF ratio for the device with the lower CNT density remains constant at 10 6 , whereas it increases from 40 to 10 5 for the device with the higher CNT density. Figure 4: Variation of property of all-carbon devices when subjected to moulding. ( a – c ) Transfer characteristics, ON and OFF currents, and mobilities of the all-carbon TFTs moulded under different conditions. The TFTs have a low-density channel, which leads to a high initial ON/OFF ratio. V DS =−0.5 V. L ch = W ch =100 μm. The currents are normalized to the same unit (A mm −1 ) because the channel dimensions increase after the moulding process. The ON and OFF currents and mobilities of 20 TFTs are plotted versus strain. The solid stars represent the median, and the upper and lower bands of the boxes correspond to the 75th and 25th percentiles, respectively, of the device population. ( d – f ) Transfer characteristics, currents and mobilities of the all-carbon TFTs moulded under different conditions. The TFTs have high-density channels, which lead to low initial ON/OFF ratios. Full size image These variations in the properties of the TFTs would be attributable to the decrease in the density of CNTs per unit area with the increase in the channel area. The increase in ON/OFF ratio of the higher-CNT-density device is caused by the density of metallic CNTs that become lower than the percolation threshold. We found no evidence to suggest that the channel CNTs are cut by the shearing force in effect at the interface between the CNTs and the surrounding polymer [31] , [32] during the forming process. The noncovalent intermolecular interactions between the CNTs and the polymer are much weaker than covalent sp [2] carbon–carbon bonds [33] , [34] , [35] . Furthermore, the shearing force decreases as the temperature increases. Because of the weak Van der Waals forces at the CNT/CNT junctions, the increase in the area of the CNT thin films is owing to the relative movements of the CNTs. In addition, the sheet resistance of CNT interconnections also increases by ∼ 60% for a strain of 18%. Demonstration of mouldable ICs The all-carbon logic ICs also exhibit mouldability. We demonstrate this by using the CNT film with the higher density for the channel to ensure that the ICs function even after being moulded. 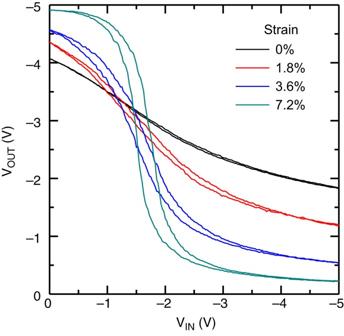Figure 5: Electrical performance of an inverter after it had been moulded. Transfer characteristics of an inverter moulded with biaxial tensile strains of 0, 1.8, 3.6 and 7.2%.VDD=−5 V. Figure 5 shows the electrical performance of a moulded inverter with various biaxial tensile strain. The ON/OFF ratio of the driving TFT of the inverter increased from 30 to 2 × 10 4 (data not shown) at a strain of 7.2%. Accordingly, the output performance of the device shows a distinct improvement, with the output voltage swings increasing from −4.0 V and −1.8 V to −4.9 V and −0.2 V, respectively, and the voltage gain from 0.8 to 11, suggesting that such logic circuits can function even after being strained to this extent. 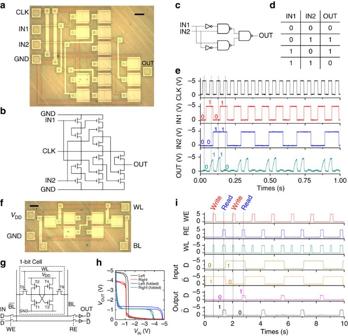Figure 6: Mouldable all-carbon ICs. (a–e) An XOR gate at a biaxial tensile strain of 7.2%. The panel includes an optical micrograph (scale bar, 100 μm), circuit symbols (diagram), truth table and input-output characteristics in response to a clock (CLK) signal. (f–i) A 1-bit SRAM device at a biaxial strain of 7.2%. (f,g) Optical micrograph (scale bar, 100 μm) and circuit diagram of the SRAM device. The two stable logic states of ‘0’ and ‘1’ are stored on four TFTs (T1, T2, T3 and T4), which form two cross-coupled inverters. Two additional access TFTs (T5 and T6) serve to control access to the storage cell during read and write operations. (h) Transfer characteristics of the two inverters measured atVDD=WL=−5 V, which are folded to show a large noise margin. (i) Write and read operation of the 1-bit SRAM atVDD=WL=−5 V. The data D andare written into the coupled inverters when ‘Write enable’ (WE) is set to ‘1’ and are stored in the SRAM even if WE becomes ‘0’. The data D andcan be read out (as shown in the bottom two panels) when ‘Read enable’ (RE) is set to ‘1’. Figure 6 shows the all-carbon ICs for an XOR gate ( Fig. 6a–e ) and an SRAM device ( Fig. 6f–i ), moulded such that they experience a 7.2% biaxial strain. The XOR gate, which represents the inequality function, consists of two inverters and three NAND gates, is operated by a clock (CLK) signal of 40 Hz and shows clear logic outputs with the large voltage swings. Figure 5: Electrical performance of an inverter after it had been moulded. Transfer characteristics of an inverter moulded with biaxial tensile strains of 0, 1.8, 3.6 and 7.2%. V DD =−5 V. Full size image Figure 6: Mouldable all-carbon ICs. ( a – e ) An XOR gate at a biaxial tensile strain of 7.2%. The panel includes an optical micrograph (scale bar, 100 μm), circuit symbols (diagram), truth table and input-output characteristics in response to a clock (CLK) signal. ( f – i ) A 1-bit SRAM device at a biaxial strain of 7.2%. ( f , g ) Optical micrograph (scale bar, 100 μm) and circuit diagram of the SRAM device. The two stable logic states of ‘0’ and ‘1’ are stored on four TFTs (T1, T2, T3 and T4), which form two cross-coupled inverters. Two additional access TFTs (T5 and T6) serve to control access to the storage cell during read and write operations. ( h ) Transfer characteristics of the two inverters measured at V DD =WL=−5 V, which are folded to show a large noise margin. ( i ) Write and read operation of the 1-bit SRAM at V DD =WL=−5 V. The data D and are written into the coupled inverters when ‘Write enable’ (WE) is set to ‘1’ and are stored in the SRAM even if WE becomes ‘0’. The data D and can be read out (as shown in the bottom two panels) when ‘Read enable’ (RE) is set to ‘1’. Full size image SRAM is a type of memory that uses bistable latching circuitry to store each bit and is faster and more reliable than dynamic RAM. To our knowledge, the present device is the first SRAM fabricated using CNT-based transistors. The 1-bit all-carbon SRAM demonstrated consists of a pair of inverters and two access transistors. The folded transfer characteristics in Fig. 6h exhibit a large noise margin for the read and write operations of the SRAM, suggesting that the SRAM operates robustly during the write and read processes. This can also be seen from the time chart in Fig. 6i . When the word line (WL) is set to ‘1’ to turn the access transistors (T5 and T6) ON, the data D and are repeatedly written or read. Other logic gates that operate similarly under a biaxial strain of 7.2% are presented in Supplementary Fig. S5 . Our demonstration of high-performance, low-voltage all-carbon TFTs and ICs opens new possibilities for transparent and flexible/stretchable electronics. Such low-voltage devices overcome the fundamental limits experienced by TFTs with 2D channels fabricated using thick polymers as insulators. This suggests that not only flexible/stretchable electronic devices but also printed ones, in which the printing of the gate insulator and low-voltage operations are usually difficult to achieve simultaneously, can be fabricated. More importantly, the mouldability of our all-carbon devices, owing to the extreme biaxial stretchability of both the passive and the active elements of the devices, could open the door for novel 3D electronic devices based on forming techniques that are used today to shape plastic products, and also allow electronic functionalities to be incorporated into plastic products at low cost. One of the major challenges that should be addressed for scaling up the CNT devices is the improvement of the performance variation of devices. The s.d. of ON current obtained in this work was σ ( I ON )/< I ON >=0.32 as shown in Supplementary Fig. S4a , which is about four time larger than that simulated for ideal random networks of CNTs with a constant length and conductivity. This suggests that the experimentally obtained variation is caused by the structural fluctuation of CNTs, and it is important to grow CNTs with a uniform length and diameter. For further improvement, metallic CNTs incorporated in the channel should be eliminated so that the density of CNTs is able to be increased without degrading ON/OFF ratio. Selective etching of metallic CNTs based on chemical [36] , electrochemical [37] , plasma [38] and light irradiation [39] methods would be applicable for present devices. Device fabrication First, metal marks (Ti/Au: 10/40 nm) were fabricated on a PEN (Teijin DuPont Films) substrate by standard photolithography, electron-beam evaporation and lift-off processes to aid in the alignment of the transparent CNT thin films. CNTs were grown using a floating-catalyst chemical vapour deposition technique and collected using a membrane filter. The dense CNT thin film for the source and drain electrodes and interconnections was transferred from the membrane filter to the substrate via a simple press transfer process [5] , and then patterned by photolithography and oxygen plasma etching processes. Next, a sparse CNT thin film to form the channels was transferred onto the substrate by dissolving the filter in acetone [9] . An insulator was formed on the substrate by spin coating a layer of PMMA (Microchem, 950 k MW) on it and baking the substrate on a hotplate at 170 °C for 1 h. The contact windows were formed by etching the PMMA insulator using acetone and a polydimethylglutarimide-based resist mask. Finally, another dense CNT film to form the gate electrodes was transferred onto the substrate and patterned using the same method as the one used to pattern the source and drain layer (See Supplementary Fig. S6 for the detail). Moulding process The fabricated all-carbon devices were fixed in the gas-moulding apparatus using screws. Compressed air at a pressure of 0.8 MPa was introduced into the moulding container, which was heated with a hotplate. After being heated for 5 min, the apparatus was allowed to cool to the room temperature, with the pressure of the compressed air being maintained. Measurements All electrical measurements were performed under ambient conditions. In order to test the logic ICs, function generators and oscilloscopes were used to generate the CLK and input signals and to observe the outputs, respectively. To prevent the input impedance of the oscilloscopes from interfering with the logic operations, high-impedance instrumental amplifiers were used as buffers. During the operation of the SRAM device, analogue switch ICs were also used to connect the bit lines to the input or output, depending ‘Write enable’ or ‘Read enable’ signals generated by a logic analyser. How to cite this article: Sun, D.-M. et al. Mouldable all-carbon integrated circuits. Nat. Commun. 4:2302 doi: 10.1038/ncomms3302 (2013).